DNA-based digital tension probes reveal integrin forces during early cell adhesion Mechanical stimuli profoundly alter cell fate, yet the mechanisms underlying mechanotransduction remain obscure because of a lack of methods for molecular force imaging. Here to address this need, we develop a new class of molecular tension probes that function as a switch to generate a 20- to 30-fold increase in fluorescence upon experiencing a threshold piconewton force. The probes employ immobilized DNA hairpins with tunable force response thresholds, ligands and fluorescence reporters. Quantitative imaging reveals that integrin tension is highly dynamic and increases with an increasing integrin density during adhesion formation. Mixtures of fluorophore-encoded probes show integrin mechanical preference for cyclized RGD over linear RGD peptides. Multiplexed probes with variable guanine-cytosine content within their hairpins reveal integrin preference for the more stable probes at the leading tip of growing adhesions near the cell edge. DNA-based tension probes are among the most sensitive optical force reporters to date, overcoming the force and spatial resolution limitations of traction force microscopy. The integrin family of transmembrane proteins constitutes one of the major force-transducing receptors in cells [1] . These receptors provide a mechanical bridge linking the extracellular matrix (ECM) to the cytoskeleton. After binding their ligands, groups of integrin receptors often nucleate the formation of focal adhesions (FAs), which are multimicron-scale structures comprised of hundreds of different adaptor and signalling proteins, such as talin, vinculin and paxillin, that take part in mechanosensing [2] . Given that the majority of integrin functions, including ligand recognition, are force modulated, it is imperative to develop approaches to report the molecular forces experienced by integrin receptors within FA assemblies [3] . Accordingly, cellular traction forces are typically imaged at the scale of FAs by using techniques that track substrate deformation, such as traction force microscopy and microfabricated post array detectors [4] , [5] , [6] , [7] . These methods underpin our current understanding of FA mechanobiology, demonstrating the existence of force oscillations and revealing the mechanotransducing role of adaptor proteins, such as vinculin [8] . However, deformable substrates alter cell biology, are either computationally intensive to use or challenging to fabricate, and ultimately hinder high-resolution imaging [9] , [10] . Moreover, the forces experienced by individual integrins are three-orders of magnitude smaller than the force sensitivity and spatial resolution of traction force microscopy and microfabricated post array detectors [11] , [12] , thus hampering more detailed elucidation of the molecular mechanisms of mechanotransduction. Genetically encoded protein tension sensors have also been developed to study the mechanoresponse of vinculin, E-cadherin and platelet endothelial cell adhesion molecule (PECAM-1) [13] , [14] , [15] , [16] . Although successful in these applications, protein engineering requires careful screening of insertion sites to ensure that localization and biological function are maintained as many proteins may not tolerate insertion of a ~500 amino-acid sequence. In addition, the optical response of genetically encoded probes is fixed to forces ranging from ~2 to ~6 pN, which is limiting given that biological forces have been estimated to exceed ~50 pN in certain processes [17] . To address these unmet needs, we invented molecular tension-based fluorescence microscopy (MTFM) to visualize pN-forces exerted by cell surface receptors, including integrin receptors [18] , [19] , [20] , [21] . In MTFM, we typically use a flexible polyethylene glycol (PEG) entropic spring that is flanked by a fluorophore-quencher pair to report cellular forces that stretch the polymer. Because the PEG-based tension probes provide a graded ‘analogue’ response from an ensemble of molecules, it is difficult to obtain the absolute magnitude of tension per receptor and to decouple this from the density of mechanically strained receptors. Dunn and colleagues tried to address this issue by using single-molecule imaging of sparsely labelled integrin tension probes (~0.5 probes per μm 2 ) [22] . Unfortunately, single-molecule imaging requires the combination of oxygen-scavengers and triplet state quenchers, which are deleterious to cells [23] , [24] . Also, the FA contains thousands of integrin receptors that dynamically transmit mechanical signals, and thus the sparse density of reporters is limiting. Wang and Ha developed tension gauge tethers, DNA duplexes that shear under sufficient force, which elegantly report minimum forces needed for receptor activation, but cannot describe the spatial and temporal dynamics of receptor activation [17] . For example, it is not clear whether the mechanical load increases per integrin molecule within the nascent adhesion, or whether the load per integrin molecule is fixed as the density of integrins increases. Ultimately, mechanical tension needs to be visualized at the level of single-integrin molecules, across a wide dynamic range of force magnitudes, and within a dynamic FA containing hundreds to thousands of receptors. To this end, we report a new class of molecular tension probes that employs a DNA hairpin as a ‘switch’ element, thus unfolding at a threshold force and reporting tension in a digital rather than analogue manner ( Fig. 1a ). DNA is ideally suited for this purpose because an oligonucleotide’s nucleobase sequence can be used to rationally tune its force-response function. Probes were designed to be highly adaptable, consisting of three oligonucleotides assembled through hybridization of 21-mer handles ( Fig. 1b ): a stem-loop DNA hairpin that is unmodified (black), a peptide-displaying ligand strand conjugated to a fluorophore (green) and a surface-anchor strand that is tagged with a quencher (blue). The apposing termini of the ligand and anchor oligonucleotides were modified with a fluorophore-quencher pair, such that a sufficient force leads to hairpin unfolding accompanied by a drastic increase in fluorescence intensity. 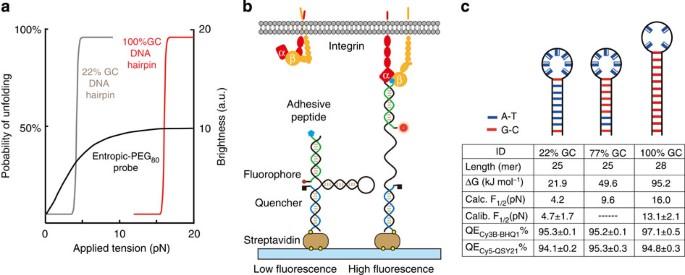Figure 1: DNA-based digital tension probes. (a) Theoretical plot showing the expected increase in fluorescence signal as a function of applied force for the 100 and 22% GC-content hairpin probes and the PEG-based tension probe. DNA-hairpin tension probe response was obtained by fitting into a two-state Boltzmann distribution. The response of the PEG-based tension probe was based on experimental parameters obtained from recent work19,21. (b) Schematic of the integrin tension sensor, which is comprised of an anchor strand immobilized onto a surface (blue), a hairpin strand that unfolds under sufficient tension (black) and a ligand strand presenting an adhesive peptide (green). At the apposing termini of the ligand and anchoring strands, a fluorophore and quencher were coupled to report the force-induced unfolding of the hairpin. (c) Schematic showing the predicted secondary structure of the folded hairpin (top). Table summarizes the calculated and measuredF1/2values, GC content and the calculated free energy of hybridization of all hairpins used in this study. The quenching efficiency (QE) for Cy3B-BHQ1 and Cy5-QSY21 fluorophore-quencher reporters was measured on supported lipid membrane and is also included in the table. Error represents the standard deviation from three different experiments. Figure 1: DNA-based digital tension probes. ( a ) Theoretical plot showing the expected increase in fluorescence signal as a function of applied force for the 100 and 22% GC-content hairpin probes and the PEG-based tension probe. DNA-hairpin tension probe response was obtained by fitting into a two-state Boltzmann distribution. The response of the PEG-based tension probe was based on experimental parameters obtained from recent work [19] , [21] . ( b ) Schematic of the integrin tension sensor, which is comprised of an anchor strand immobilized onto a surface (blue), a hairpin strand that unfolds under sufficient tension (black) and a ligand strand presenting an adhesive peptide (green). At the apposing termini of the ligand and anchoring strands, a fluorophore and quencher were coupled to report the force-induced unfolding of the hairpin. ( c ) Schematic showing the predicted secondary structure of the folded hairpin (top). Table summarizes the calculated and measured F 1/2 values, GC content and the calculated free energy of hybridization of all hairpins used in this study. The quenching efficiency (QE) for Cy3B-BHQ1 and Cy5-QSY21 fluorophore-quencher reporters was measured on supported lipid membrane and is also included in the table. Error represents the standard deviation from three different experiments. Full size image Because each probe engages only a single receptor, the signal intensity from an ensemble of digital tension reporters is linearly proportional to the number of integrin molecules exceeding a threshold force. This relationship overcomes the challenges of inferring single-receptor forces from an ensemble fluorescence measurement; that is, de-convoluting the relationship between probe density and the magnitude of tension per probe. Therefore, these reversible DNA-based probes obviate the need for estimating the average minimum force per receptor [18] , [19] , [20] , [21] or conducting single-molecule measurements [22] . Design and synthesis of DNA-based tension probes We synthesized a small library of hairpin sensors with different GC contents, stem lengths and loop sizes to tune their stability and their F 1/2 , the force at which 50% of hairpins unfold ( Fig. 1c , Methods, Supplementary Figs 1 and 2 , Supplementary Tables 1 and 2 , Supplementary Note I ). The value of F 1/2 was initially estimated using the free energy of hairpin unfolding at zero force, as well as the free energy required to stretch single-strand DNA (ssDNA) based on the worm-like chain model (Methods, Supplementary Table 3 , Supplementary Note II ) [25] , [26] . 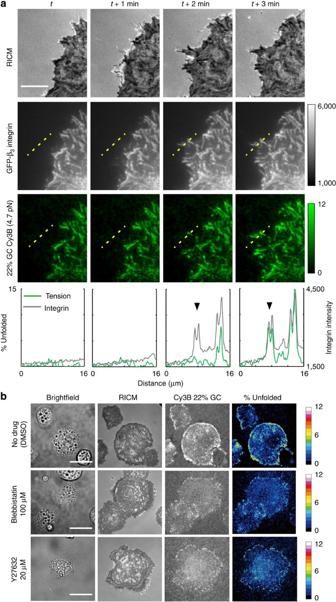Figure 3: Control experiments show that tension sensor response is mechanically mediated by integrin receptors. (a) Co-localization of the integrin tension signal with GFP-β3-integrin fluorescence. Rat embryonic fibroblast (REF) cells transfected with GFP-β3-integrin were plated on a surface that encoded the 22% GC content probe with Cy3B. The images show RICM, GFP and Cy3B channels acquired over four time points. The intensity of the Cy3B channel corresponds to the fraction of 22% GC content hairpins that were unfolded under the cell. Linescan analysis of the two fluorescence channels is shown below each time point and show the arrival of the integrin receptors followed by the increase of integrin tension. This indicates that the majority of observed tension signal is transduced through the β3-integrin receptor. Scale bar, 10 μm. (b) Blocking myosin II activity modulates integrin mechanical tension during initial cell spreading and adhesion. Representative images in brightfield, RICM and Cy3B channels for control cells as well as cells treated with myosin II inhibitors blebbistatin and the ROCK inhibitor Y27632. The fourth column of images represents the fraction of 22% GC hairpins unfolded under tension and is quantified using a colour-coded heat map. Images were acquired 20 min after cell seeding on cRGDfK-modified tension probes. Scale bar, 10 μm. The 22 and 100% GC content probes were further calibrated by using the biomembrane force probe (BFP), which is a single-molecule force spectroscopy technique based on optically monitoring the displacement of the interface between a microparticle and a red blood cell (RBC) [27] . Using a loading rate of 500 pN s −1 , we found that the experimental F 1/2 of the 22 and 100% GC probes was 4.7±1.7 pN ( n =36 unfolding events) and 13.1±2.4 pN ( n =63 unfolding events), respectively (Methods and Supplementary Fig. 3 ). Note that although the calculated and experimentally determined F 1/2 values generally agree, there is a greater difference for the larger sized hairpins. Also, broadening of the unfolding probability compared with the expected Boltzmann distribution is likely due to thermal noise and the heterogeneity in the orientations of the molecules probed. To identify the most sensitive fluorescent reporters, a series of probes with different fluorophore-quencher pairs were synthesized and characterized to determine the quenching efficiency (QE) at 37 °C in PBS. We found that Cy3B-BHQ1, Atto647N-QSY21 and Cy5-QSY21 showed the greatest QEs (~95%) among the dye-quencher pairs tested, and fully recover their fluorescence upon opening the hairpin with a complementary DNA strand ( Fig. 1c , Methods, Supplementary Fig. 4 , Supplementary Table 4 ). 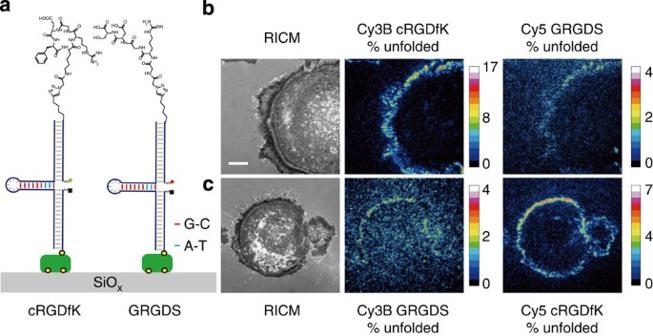Figure 4: Integrin mechanical response specificity using spectrally encoded hairpin probes presenting different ligand types. (a) Schematic of multiplexed tension probes modified with cyclic RGDfK and linear GRGDS peptides that were coupled to sensors employing identical hairpins (77% GC content), and encoded using different fluorophore-quencher reporters. (b) Representative RICM and % unfolded maps for cells cultured on substrates shown ina. The fluorophore-quencher encoding was reversed incto exclude potential imaging artifacts. Inbandc, at least a twofold greater population of cyclic RGDfK peptide sensors were unfolded compared with the linear GRGDS peptides. Scale bar, 10 μm. Importantly, these QE values (95–97%) are greater than those reported for any molecular tension probe, yielding a 20- to 30-fold increase in signal over background, which represents a two- to threefold improvement over PEG-based entropic spring reporters ( Fig. 1a ) [18] , [19] , [20] , [21] . Visualizing integrin tension The DNA surface density on glass coverslips was empirically tuned (~400 molecules per μm 2 , Methods and Supplementary Fig. 5 ) to support cell adhesion while limiting the background fluorescence. Breast cancer cells (HCC1143) were plated onto the 22% GC ( F 1/2 =4.7 pN) hairpin probe surface displaying cyclic Arg-Gly-Asp- D -Phe-Lys (cRGDfK) and then timelapse videos were acquired as cells initiated spreading and adhesion ( Fig. 2 and Supplementary Movie 1 ). Initially, the tension signal was diffuse and included puncta of higher intensity. Within minutes, the tension signal localized to the cell edges and rapidly increased in intensity (up to 9% of probes were unfolded), which indicated that a larger density of hairpins were ruptured at those regions (force ≥4.7 pN). We determined the percentage of unfolded tension probes by calculating the fluorescence intensity of de-quenched dye corresponding to a fully opened hairpin probe, and assuming a linear relationship between the fraction of hairpins unfolded and the fluorescence intensity (Methods, Supplementary Figs 6 and 7 , Supplementary Tables 5–9 ). Linescan analysis shows the progression of cellular forces across three nascent adhesions over a 5-min time period ( Fig. 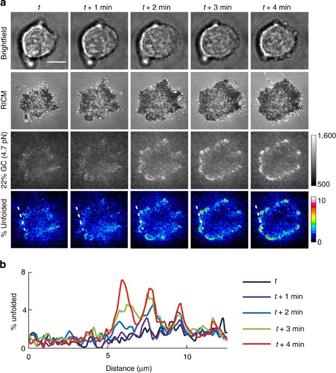2 ). This timelapse sequence shows that cell adhesion forces are highly dynamic, heterogeneous and rapidly exceed the estimated 4.7 pN F 1/2 during initial cell spreading. Figure 2: Visualizing integrin tension with DNA-based MTFM probes. (a) Representative brightfield, RICM and MTFM (22% GC content hairpin probe) timelapse images at the indicated time points showing the initial stage of cell spreading and adhesion. The intensity of the 22% GC probe channel is in raw arbitrary units. The % unfolded channel indicates the fraction of the 22% GC hairpins that have been unfolded within each pixel. (b) Linescan analysis plot of the region highlighted with dashed white line inashows the dynamic growth of tension within three growing adhesions. Scale bar, 10 μm. Figure 2: Visualizing integrin tension with DNA-based MTFM probes. ( a ) Representative brightfield, RICM and MTFM (22% GC content hairpin probe) timelapse images at the indicated time points showing the initial stage of cell spreading and adhesion. The intensity of the 22% GC probe channel is in raw arbitrary units. The % unfolded channel indicates the fraction of the 22% GC hairpins that have been unfolded within each pixel. ( b ) Linescan analysis plot of the region highlighted with dashed white line in a shows the dynamic growth of tension within three growing adhesions. Scale bar, 10 μm. Full size image To confirm that hairpin unfolding is mechanically mediated through integrin receptors, we plated rat embryonic fibroblasts expressing GFP-β 3 -integrin on 22% GC probe surface ( Fig. 3a ). Timelapse total internal reflection fluorescence microscopy showed tension signal co-localization with GFP, confirming that forces were primarily exerted through the β 3 integrin receptors [28] , [29] , and that tension increases following recruitment of β 3 -integrin. Treatment of cells with latrunculin B, an inhibitor of actin polymerization, led to complete and rapid (1–3 min) decay of the tension signal, confirming that the signal is reversible and F-actin dependent ( Supplementary Movie 2 ). In contrast, myosin II inhibition using blebbistatin or the ROCK inhibitor, Y27632, did not abolish integrin tension, but led to a lower density of unfolded probes ( Fig. 3b ). Control experiments in which cells were seeded onto RGD-lacking DNA probes, either with or without the hairpin structure, did not show any cell attachment or sensor activation ( Supplementary Fig. 8a,b ). Importantly, cells plated on a binary mixture of DNA sensors, one that lacked the RGD peptide, whereas the second lacking the dye-quencher pair, showed that the cells spread but failed to generate a fluorescence response ( Supplementary Fig. 8c ). Together, these results unambiguously demonstrate that hairpin probes report integrin-specific and cytoskeletal-mediated forces. Figure 3: Control experiments show that tension sensor response is mechanically mediated by integrin receptors. ( a ) Co-localization of the integrin tension signal with GFP-β 3 -integrin fluorescence. Rat embryonic fibroblast (REF) cells transfected with GFP-β 3 -integrin were plated on a surface that encoded the 22% GC content probe with Cy3B. The images show RICM, GFP and Cy3B channels acquired over four time points. The intensity of the Cy3B channel corresponds to the fraction of 22% GC content hairpins that were unfolded under the cell. Linescan analysis of the two fluorescence channels is shown below each time point and show the arrival of the integrin receptors followed by the increase of integrin tension. This indicates that the majority of observed tension signal is transduced through the β 3 -integrin receptor. Scale bar, 10 μm. ( b ) Blocking myosin II activity modulates integrin mechanical tension during initial cell spreading and adhesion. Representative images in brightfield, RICM and Cy3B channels for control cells as well as cells treated with myosin II inhibitors blebbistatin and the ROCK inhibitor Y27632. The fourth column of images represents the fraction of 22% GC hairpins unfolded under tension and is quantified using a colour-coded heat map. Images were acquired 20 min after cell seeding on cRGDfK-modified tension probes. Scale bar, 10 μm. Full size image At later time points (~40 min) following cell seeding, we found that the fluorescence intensity under cells decreased to levels below that of the quenched sensor background, for both cyclic and linear RGD ligand ( Supplementary Fig. 9 ). This loss in fluorescence was mainly due to force-induced dissociation of the ligand strand ( Supplementary Fig. 10 ), rather than nuclease activity, or biotin-streptavidin dissociation, as observed with PEG-based MTFM probes [20] . Shearing of the fluorescent ligand-presenting strand is in agreement with recent results obtained using tension gauge tethers [17] . Although ligand strand shearing at later time points simply reduces fluorescence and does not lead to false positive signal, the current probe design is better suited for imaging early FA mechanics, and for imaging weaker receptor-mediated forces such epidermal growth factor endocytosis and Notch activation [17] , [18] , [30] . Selective mechanical response toward linear and cyclic RGD Given the molecular specificity of these probes, we next wondered whether integrin receptors would display mechanical selectivity when presented with a mixture of ligands. This is an important question because the ECM is comprised of nanoscale fibrillar protein assemblies that are chemically heterogeneous. For example, conventional techniques such as traction force microscopy report the average nN force from micrometre-sized elements, thus obscuring molecular specificity of tension in a complex mixture of ECM ligands [4] . We generated cRGDfK- and linear GRGDS-modified tension probes that were spectrally encoded by Cy3B-BHQ1 and Cy5-QSY21 reporters, respectively ( Fig. 4 ). Both ligand strands were hybridized to the 77% GC content sensors and anchored to a substrate in 1:1 molar ratio. Cells plated onto this multiplexed surface generated signals that were highly localized at the lamella in the two fluorescence channels ( Fig. 4b ). However, the intensity of the linear peptide channel was significantly weaker, and showed at least a twofold smaller number of unfolded hairpins when compared with cRGDfK ligands and also when compared with the signal generated by surfaces exclusively presenting the linear GRGDS 77% GC content sensor ( Supplementary Fig. 11 ). To exclude the possibility that this difference was due to fluorophore photophysics and other artefacts ( Supplementary Figs 12–14 ), we swapped the dye-quenchers pair encoding and observed the same trend ( Fig. 4c ). These results show that integrin-ligand mechanical selectivity acts at the individual ligand level, whereby RGD ligand variants experience differential magnitudes of tension regardless of their spatial proximity. The mechanism for this selectively is likely due to lower integrin affinity for linear RGD ligands when compared with cyclic RGD peptides [28] . These results demonstrate how integrin receptors would mechanically respond when presented with chemically heterogeneous ECM ligands in more physiologically relevant settings. Figure 4: Integrin mechanical response specificity using spectrally encoded hairpin probes presenting different ligand types. ( a ) Schematic of multiplexed tension probes modified with cyclic RGDfK and linear GRGDS peptides that were coupled to sensors employing identical hairpins (77% GC content), and encoded using different fluorophore-quencher reporters. ( b ) Representative RICM and % unfolded maps for cells cultured on substrates shown in a . The fluorophore-quencher encoding was reversed in c to exclude potential imaging artifacts. In b and c , at least a twofold greater population of cyclic RGDfK peptide sensors were unfolded compared with the linear GRGDS peptides. Scale bar, 10 μm. Full size image F 1/2 -encoded probes to analyze force distribution within FAs To analyze the spatial distribution of forces within individual growing adhesions, we spectrally encoded a binary mixture of cRGDfK tension probes with the 100 and 22% GC hairpins using the Atto647N and Cy3B dyes ( Fig. 5a ). As expected, cells attached and spread onto this 1:1 ratio multiplexed sensor surface, generating similar signals in both fluorescence channels ( Fig. 5a and Supplementary Movie 3 ). Timelapse imaging showed that both probes displayed similar dynamics, spatial localization and intensities (unfolding percentage per unit area) during cell spreading and FA formation ( Fig. 5a–c ). This trend was maintained when the encoding was swapped ( Supplementary Movie 4 ) or when both channels were encoded using the same 100% GC content probe. This general agreement between the two channels indicates that most engaged integrin receptors exerted tension that was greater than or equal to 13.1 pN. 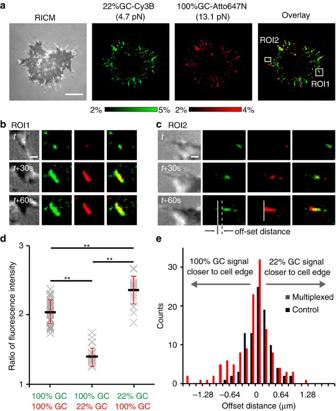Figure 5: Investigating the force distribution within integrin clusters using spectrally encoded tension probes with differentF1/2. (a) Representative RICM and % unfolded maps of the 22% GC hairpin probe (Cy3B-BHQ1, green), 100% GC hairpin probe (Atto647N-QSY21, red) and the overlay channel of a single cell during initial spreading. A ~30-min duration timelapse video of these channels is included asSupplementary Movie 3. Scale bar, 10 μm. Note thatSupplementary Movie 4shows a timelapse movie collected using similar experimental conditions but using the reversedF1/2-fluorophore encoding to that used inSupplementary Movie 3. (b) Zoom-in of region of interest 1 (ROI1) showing the dynamics of a growing adhesion where the 22% GC probe signal was greater than that of the 100% GC probe. Scale bar, 2 μm. (c) Zoom-in of ROI2 showing the dynamics of a growing adhesion where the start point of the adhesion appeared closer to the cell edge in the 100% GC probe channel compared with the 22% GC probe channel (offset). Scale bar, 2 μm. (d) Plot showing the ratio of the intensities of the Cy3B and Atto647 fluorescence channels when the encoding was as follows: Cy3B-100% GC and Atto647N-100% GC; Cy3B-100% GC and Atto647N-22% GC; Cy3B-22% GC and Atto647N-100% GC. The data were collected fromn=15 cells, error bars represent the standard error of the mean (s.e.m.).Supplementary Fig. 15details how the data were analyzed. **P-value <0.01 int-test. (e) Histogram analysis of the offset between the 100% GC and 22% GC hairpin probe signal at the cell edge (221 adhesions fromn=17 cells). Data analysis is described inSupplementary Figs 16 and 17. The black bars represent the control where both channels were encoded using the 100% GC hairpin, whereas the red bars represent experiments where each channel encoded either the 100 or 22% GC probes. The control histogram was best fit using a single Gaussian peak, whereas the multiplexed histogram was best fit to two Gaussian peaks. Figure 5: Investigating the force distribution within integrin clusters using spectrally encoded tension probes with different F 1/2 . ( a ) Representative RICM and % unfolded maps of the 22% GC hairpin probe (Cy3B-BHQ1, green), 100% GC hairpin probe (Atto647N-QSY21, red) and the overlay channel of a single cell during initial spreading. A ~30-min duration timelapse video of these channels is included as Supplementary Movie 3 . Scale bar, 10 μm. Note that Supplementary Movie 4 shows a timelapse movie collected using similar experimental conditions but using the reversed F 1/2 -fluorophore encoding to that used in Supplementary Movie 3 . ( b ) Zoom-in of region of interest 1 (ROI1) showing the dynamics of a growing adhesion where the 22% GC probe signal was greater than that of the 100% GC probe. Scale bar, 2 μm. ( c ) Zoom-in of ROI2 showing the dynamics of a growing adhesion where the start point of the adhesion appeared closer to the cell edge in the 100% GC probe channel compared with the 22% GC probe channel (offset). Scale bar, 2 μm. ( d ) Plot showing the ratio of the intensities of the Cy3B and Atto647 fluorescence channels when the encoding was as follows: Cy3B-100% GC and Atto647N-100% GC; Cy3B-100% GC and Atto647N-22% GC; Cy3B-22% GC and Atto647N-100% GC. The data were collected from n =15 cells, error bars represent the standard error of the mean (s.e.m.). Supplementary Fig. 15 details how the data were analyzed. ** P -value <0.01 in t -test. ( e ) Histogram analysis of the offset between the 100% GC and 22% GC hairpin probe signal at the cell edge (221 adhesions from n =17 cells). Data analysis is described in Supplementary Figs 16 and 17 . The black bars represent the control where both channels were encoded using the 100% GC hairpin, whereas the red bars represent experiments where each channel encoded either the 100 or 22% GC probes. The control histogram was best fit using a single Gaussian peak, whereas the multiplexed histogram was best fit to two Gaussian peaks. Full size image Upon closer inspection of the data, we noted two additional features. The first was that a subset of FAs appeared larger and more intense in the 22% GC probe channel than the 100% GC probe channel ( Fig. 5b ). To quantify this observation, we measured the ratio of the signal intensity when the 100 and 22% GC content probes were encoded with Atto647N and Cy3B, respectively, and compared this to experiments with reversed encoding as well as control experiments where both probes used the 100% GC hairpin ( Fig. 5d , n =15 cells; Supplementary Fig. 15 ). This confirms that a subset of integrins exert tension that is lower than 13.1 pN but greater than 4.7 pN. The existence of such a subpopulation is expected, as the tension must gradually rise per integrin during FA maturation. The second observation was that a subset of FAs near the cell edge preferentially triggered the 100% GC probe over the 22% GC probe specifically at the tips of these adhesions ( Fig 5c and e ). To verify the statistical significance of this observation, we measured the offset between the start positions of tension signal in the two fluorescence channels when each channel encoded different hairpins and when each channel encoded the same 100% GC hairpin (as a control). Histogram analysis of 221 adhesions from 17 cells indicated that there is a subset of FAs where the 100% GC hairpin probe was triggered ~0.5 μm ahead of the 22% GC probe ( Fig. 5e , and Supplementary Figs 16 and 17 ). This small population of FAs with an offset is not observed in the control experiment and is counterintuitive, as both probes are chemically identical and the 22% GC probes mechanically denature at significantly lower forces than the 100% GC probes. Thus, one would expect to observe the opposite phenomenon, that is, the 22% GC probe should be triggered closer to the cell edge because the integrin-ligand association rates are identical for both probes and initial adhesions likely exert lower magnitude forces that may not be sufficient to trigger the 100% GC content probes. Therefore, the offset in the start position of tension indicates that there is a small differential preference for integrins to remain bound to the more rigid 100% GC probes that can support higher forces before yielding, thus suggesting a molecular basis for cellular rigidity sensing of the substrate. Although further work is needed to fully elucidate the molecular underpinnings of the observed preference, the results obtained from multiplexed sensors highlight the unique capabilities of DNA-tension probes, providing a new approach to investigate differential integrin forces in a manner dependent on chemomechanical properties of individual ligand molecules. DNA-based tension probes confer several advantages. First, the predictable secondary structure places the fluorophore-quencher pair in a well-defined position, thus lowering background signal and increasing the signal-to-noise ratio (~20- to 30-fold over background). This design strategy is widely used by molecular beacon-based assays [31] . Accordingly, the F 1/2 is highly tailorable, and the hairpin can be precisely tuned to generate a clear binary response at a desired threshold tension (~1–20 pN) [25] . Second, by employing a three-strand system, we circumvent chemical modification of the hairpin oligonucleotide, and therefore, existing models can be used to estimate the F 1/2 . The three-strand design is also advantageous because it allows one to tune libraries of F 1/2 values while avoiding re-synthesis of the anchor and ligand strands. In principle, the anchoring strand (and DNA-probes) can be attached to virtually any type of material, including three-dimensional matrices that better mimic the ECM, which is of great interest to the community. The caveat of the three-strand design pertains to force-induced shearing of the probe from the surface, which is a unique problem associated with the large mechanical loads in integrin-based mechanotransduction processes. Third, although an ensemble of DNA tension probes are engaged and activated within each diffraction limited region, which is necessary to support cell adhesion, we extract molecular details because each sensor functions as a digital switch for well-defined thresholds of force. Finally, the growing availability of inexpensive and rapid oligonucleotide synthesis allows one to easily generate and systematically test libraries of tension probes with tunable force sensitivity, thus ensuring the broad dissemination of this method. DNA-based tension probes All oligonucleotides were custom synthesized and purified by Integrated DNA Technologies, unless otherwise noted. This design consisted of a ssDNA hairpin hybridized through two 21-mer DNA handles to the ligand and anchor strands ( Supplementary Table 1 ). Poly(T) was used for the hairpin loop sequence to avoid secondary structures and base stacking. The 3′ terminus of the anchor strand was modified with a biotin group to immobilize the oligonucleotide to a streptavidin surface. The alkyne group at the 5′ terminus of the ligand strand was used in a 1′,3′ dipolar cycloaddition click reaction to couple the appropriate RGD peptides. To generate multiplexed tension probe surfaces, each hairpin sensor was folded separately and then mixed at 1:1 ratio and added to the streptavidin surface. F 1/2 calculation for DNA hairpin The following F 1/2 calculation was primarily based on the assumptions and measurements used by Woodside et al. [25] The total free energy of the hairpin can be described as follows: where ΔG fold is the free energy of unfolding the hairpin at F =0, F is the externally exerted force, x is the hairpin extension and ΔG stretch is the free energy of stretching the ssDNA from F =0 to F = F 1/2 , and can be calculated from worm-like chain model as follows [25] : where L p is the persistence length of ssDNA (~1.3 nm), L 0 is the contour length of ssDNA (~0.63 nm per nucleotide), x is the hairpin extension from equilibrium and was calculated by using (0.44 × ( n - 1 )) nm, and k B is the Boltzmann constant and T is temperature. To use these equations and estimate the F 1/2 for each hairpin probe, we determined the sum of ΔG fold and ΔG stretch , and estimated the hairpin displacement needed for unfolding, Δx , by using ((0.44 × ( n - 1 ))-2) nm, where n represents the number of bases comprising the hairpin. Note that we subtract a distance of 2 nm because this corresponds to the initial separation between the hairpin termini, which is set by the diameter of the hairpin stem duplex (effective helix width) [25] . When F = F 1/2 , then the free energy of the transition equals zero and the F 1/2 can be rearranged as follows: In our calculations, ΔG stretch was determined using Supplementary Equation 2 without modification. ΔG fold was determined using nearest neighbour free energy parameters obtained from the IDT oligoanalyzer 3.1, which uses the UNAfold software package, and will now be referred to as ΔG IDT . Equation (3) was used to infer the F 1/2 for tension probes at experimental conditions (37 °C, 140.5 mM Na + and 0.4 mM Mg 2+ ), and these data are summarized in Supplementary Table 3 . Force probes calibration by BFP The BFP measurement was based on previous work, which has been described in detail elsewhere [27] . In the BFP setup, a biotinylated RBC was first aspirated by a micropipette. A streptavidinylated glass bead was then attached to the apex of the RBC to form an ultra-sensitive force probe. On the opposite side, a bead coated with our DNA force probe was aspirated by a target micropipette. A piezoelectric translator (Physical Instrument) drove the target pipette with sub-nanometer precision via a capacitive sensor feedback control. The beads were assembled in a cell chamber filled with L15 media supplemented with 5 mM HEPES and 1% BSA and observed under an inverted microscope (Nikon TiE, Nikon) through two cameras. One camera (GC1290, Procilica) captured real-time images at 30 frames per second (f.p.s. ), whereas the other (GE680, Proscilica) recorded at 1,600 f.p.s. as the region of interest was confined to the contact interface between the RBC and the bead. A customized LabView (National Instrument) programme analyzed the image and tracked in real time the position of the bead with a 3-nm displacement precision [32] . The BFP spring constant was set to ~0.3 pN nm −1 , and it was determined from the suction pressure inside the probe pipette that held the RBC, the radius of the probe pipette, the diameter of the spherical portion of the RBC outside of the pipette and the contact area between the RBC and the probe bead [32] , [33] . Briefly, in a measurement cycle, a DNA-coated 5-μm silica bead was brought into contact with the probe bead with a 20-pN impingement force for 0.1 s to allow bond formation. The target pipette was then retracted at 500 pN s −1 until it reached a 20-pN force level before dropping the force level to ~0 pN by bringing the two beads into close proximity again. The biotin-streptavidin bond was ruptured after 1 s, and the target bead was returned to the original position to start the next cycle. To ensure that most adhesion events were due to single bonds, adhesion frequency (number of adhesions divided by total number of contacts) was controlled to be ≤20% by adjusting the coating density of the DNA force probe [34] . An unfolding event was identified by a dip in force level in the force-ascending phase ( Supplementary Fig. 3a ), because of the lengthening of the DNA upon hairpin opening. Similarly, a folding event was identified by a rise in force level in the force-descending phase. The force at which each unfolding event occurred was recorded and the cumulative histogram was plotted in Supplementary Fig. 3 to determine the F ½ . QE measurement for different reporter pairs To identify the optimal fluorophore-quencher pairs for the DNA-based MTFM probes, we synthesized a series of probes with different reporters and measured their QE ( Supplementary Table 4 ). MTFM probes were anchored to supported lipid membrane, to minimize nonspecific binding and ensure a homogeneous and reproducible DNA density across all the tested pairs. Fluorophore labelling was performed as described in Supplementary Note 1 and associated text. For all these measurements, a 45-mer hairpin (H45, ~15.38 nm, Supplementary Table 1 ) was used to ensure that the donor was completely dequenched upon hybridization. The fluorescence intensity of the hairpin sensor, I DA , was measured with the closed H45 in triplicate ( Supplementary Fig. 4 ). To measure the donor only intensity, I D , H45 was hybridized to a complementary strand (tenfold molar excess), and then assembled with the DNA handles and anchored to the surface. Based on these measurements, we selected the Cy5-QSY21, Atto647N-QSY21 and Cy3B-BHQ1 pairs given their superior QE when compared with other fluorophore quencher combinations. Calibration curve and determination of F factor and sensor density This protocol has been adapted from Galush et al. [35] , and is briefly described in this section. To calibrate the fluorescence intensity, 1,2-dioleoyl- sn -glycero-3-phosphocholine (DOPC)-supported lipid membranes were doped with TRITC-DHPE lipids with concentrations ranging from 0 to 0.08 mol% and imaged under the same conditions used in live cell imaging ( Supplementary Fig. 5 ). The number of fluorophore molecules per unit area was estimated from the footprint of DOPC, which was reported at 0.72 nm 2 . To use the calibration curve, the intensity of the ligand molecules was compared with the lipid-fluorophore standards to obtain the F factor. The F factor is defined as: , where I bulk(sensor) and I bulk(TRITC-DHPE) are the intensity of the ligand or lipid molecules in solution after being normalized for concentration. This value was measured on the fluorescence microscope by moving the focal plane (~200 μm) into the centre of the sample. Measurement of QE (1- I DA /I D ) on glass substrate To determine the QE as a function of the hairpin used in DNA-based tension probes, we recorded the fluorescence intensity of the closed hairpin, I DA , on glass substrates at experimental conditions (37 °C, cell media; Supplementary Fig. 6a, c ). To measure the donor only intensity, I D , tension probes were hybridized to their complementary strands (tenfold molar excess) and DNA handles ( Supplementary Fig. 6b, d ). Note that these QE value were in general agreement with the values obtained on supported lipid membranes in 1 × PBS at room temperature. Conversion of I DA / I D to calculate the fraction of unfolded hairpins To calculate the fraction of hairpins that are unfolded from any given cell experiment, we assumed that the fluorescence intensity of immobilized tension probes at resting ( F =0 pN) corresponded to a monolayer of fully folded hairpins (0% unfolded, I DA ). As hairpins that were hybridized with a tenfold excess of complementary stands are completely dequenched ( Supplementary Fig. 4 ), the fluorescence intensity from this surface corresponds to hairpins that are 100% unfolded. Therefore, the fluorescence intensity of the 100% unfolded hairpins corresponds to I D . Given that there is a linear relationship between the fraction of unfolded hairpins and the QE, we used the ratio of I DA / I D to obtain this linear function ( Supplementary Fig. 6e ). This linear relationship was then used to convert the fluorescence intensity from the cell experiment to the fraction of unfolded hairpins (% unfolded). Imaging parameters Supplementary Tables 5–9 summarize all the imaging parameters used in our experiments. Sensors with GC content of 22% and 77% GC have the same length (25mer); therefore, these two sensors share the same values for QE, I DA / I D and conversion function, which were determined from the 77% GC probe surface. We assumed that the QE for each probe remained the same regardless of whether it was displayed in single-channel experiment or if it was included as part of a multiplexed surface with hairpins of different F 1/2 . Surface preparation The glass substrates were covalently functionalized with biotin and modified with streptavidin by using previously published literature procedures [18] . Briefly, glass coverslips (number 2, 25-mm diameter; VWR) were sonicated in Nanopure water for 10 min and then etched in piranha (a 3:1 mixture of sulfuric acid (Avantor Performance Materials) and hydrogen peroxide (Sigma)) for 10 min (please take caution: piranha is extremely corrosive and may explode if exposed to organics). The glass coverslips were then washed six times in a beaker of Nanopure water (18.2 mω) and placed into three successive wash beakers containing EtOH (Decon Labs) and left in a final fourth beaker containing 1% (3-aminopropyl)triethoxysilane (Sigma) in EtOH for 1 h. The substrates were then immersed in the EtOH three times and subsequently rinsed with EtOH and dried under nitrogen. Substrates were then baked in an oven (~100 °C) for 10 min. After cooling, the samples were incubated with NHS-biotin (Thermo Fisher) at 2 mg ml −1 in dimethyl sulfoxide (Sigma) overnight. Subsequently, the substrates were washed with EtOH and dried under nitrogen. The substrates were then washed with 1 × PBS (3 × 5 ml) and incubated with BSA (EMD Chemicals, 100 μg μl −1 , 30 min) and washed again with 1 × PBS (3 × 5 ml). Streptavidin was then added (1 μg ml −1 45 min, room temperature) followed by washing with 1 × PBS (3 × 5 ml). The chambers were then incubated with the DNA-based tension sensor (10 nM) for 1 h and rinsed before conducting cell experiments and imaging. Supported lipid membrane preparation The supported lipid bilayers were prepared by mixing 99.9% DOPC and 0.1% 1,2-dioleoyl- sn -glycero-3-phosphoethanolamine-N-(cap biotinyl) (sodium salt) (DPPE-biotin). The solution was dried with a rotary evaporator and placed under a stream of N 2 to ensure complete evaporation of the solvent. These lipid samples were then resuspended in Nanopure water and subjected to three freeze/thaw cycles by alternating immersions in an acetone and dry ice bath and a warm water bath (40 °C). To obtain small unilamellar vesicles, lipids were extruded through a high-pressure extruder with a 200-nm nanopore membrane (Whatman). Supported lipid bilayers were assembled by adding small unilamellar vesicle’s to 1 M NaOH-etched 96-well plates with glass-bottomed wells. After blocking with 0.1% BSA for 30 min, bilayer surfaces were incubated with streptavidin (1 μg per 400 μl) for 1 h. Wells were rinsed three times with 5 ml of 1 × PBS, then incubated with the appropriate DNA hairpin sensors duplex (50 nM) for 1 h and rinsed 3 × with 5 ml of 1 × PBS before imaging. High-performance liquid chromatography All DNA conjugates were purified by using a C18 column (diameter: 4.6 mm; length: 250 mm) in a reverse phase binary pump high-performance liquid chromatography that was coupled to a diode array detector (Agilent 1100). The flow rate was generally set to 1 ml min −1 with a linear gradient of 10–60% B over 50 min (A: aqueous 0.1 M triethylammonium acetate buffer; B:acetonitrile (LC-MS Chromasolv, ≥99.9%; Fluka)). Unless otherwise noted, this elution gradient was followed by a second gradient of 60–100% B over 10 min to collect the more hydrophobic fractions. Matrix-assisted laser desorption/ionization (MALDI)-time-of-flight mass spectroscopy The matrix was prepared by dissolving 20 mg 3-hydroxypicolinic acid into 1 ml of matrix solvent (50% acetonitrile, 0.1% trifluoroacetic acid and 10% of a solution of 50 mg ml −1 ammonium citrate). 2 μl of this mixture was added to each well on the MALDI plate. After allowing the solution to dry for 20 min, the sample was analyzed by a high-performance MALDI time-of-flight mass spectrometer (Voyager STR). Fluorescence microscopy Live cells were imaged in standard cell media at 37 °C, and fixed cells were imaged in 1% BSA in 1 × PBS at room temperature. During imaging, physiological temperature was maintained with a warming apparatus consisting of a sample warmer and an objective warmer (Warner Instruments, 641674D and 640375). The microscope was a Nikon Eclipse Ti driven by the Elements software package. The microscope features an Evolve electron multiplying charge-coupled device (Photometrics), an Intensilight epifluorescence source (Nikon), a CFI Apo × 100 (numerical aperture=1.49) objective (Nikon) and a TIRF launcher with two laser lines: 488 nm (10 mW) and 638 nm (20 mW). This microscope also includes the Nikon Perfect Focus System, an interferometry-based focus lock that allowed the capture of multipoint and time-lapse images without loss of focus. The microscope was equipped with the following Chroma filter cubes: TIRF 488, TRITC, Epi 640 and reflection interference contrast microscopy (RICM). Hairpin hybridization All DNA oligonucleotides were allowed to fold into their hairpin secondary structure in 50 μl PBS at a concentration of 100 nM in a 0.2-ml Thermowell Tube . All oligonucleotides were first denatured at 75 °C for 5 min. This was followed by a renaturation step in which the temperature was allowed to return to room temperature at a rate of 1.3 °C min −1 . Cell culture HCC1143 human breast carcinoma cells were cultured in RPMI 1640 medium (Mediatech) supplemented with 10% FBS (Mediatech), HEPES (9.9 mM, Sigma), sodium pyruvate (1 mM, Sigma), L-glutamine (2.5 mM, Mediatech), penicillin G (100 IU ml −1 , Mediatech) and streptomycin (100 μg ml −1 , Mediatech) and were incubated at 37 °C with 5% CO 2 . Cells were passaged at 90% confluency and plated at a density of 50% and media renewed every 3 days. NIH 3T3 mouse embryonic fibroblasts and rat embryonic fibroblasts expressing GFP-β 3 -integrin cells were cultured in DMEM (Mediatech) supplemented with 10% Calf Serum (Mediatech), L-glutamine (2.5 mM, Mediatech), penicillin G (100 IU ml −1 , Mediatech) and streptomycin (100 μg ml −1 , Mediatech) at 37 °C with 5% CO 2 . Cells were passaged at 80% confluency and plated at a density of 4 × 10 3 cells per cm 2 (100 × 10 3 cells per flask) and media renewed every 3 days. Reagents The fluorescent dye Cy5 NHS ester (Cat. # 23020) was purchased from Lumiprobe corporation. The fluorescent dye Cy3B NHS ester (Product code: PA63101) was purchased from GE Healthcare Life Science. Quencher QSY21 succinimidyl ester (Cat. # Q-20132) was purchased from Life Technologies. The fluorescent dye Atto 647N NHS ester was purchased from Sigma-Aldrich. Cyclo [Arg-Gly-Asp-d-Phe-Lys(PEG-PEG)] (Product code: PCI-3696-PI, c(RGDfK(PEG-PEG)), PEG=8-amino-3,6-dioxaoctanoic acid) was acquired from Peptides International. Gly-Arg-Gly-Asp-Ser (Cat. # G4391) was purchased from Sigma-Aldrich. Glass coverslips (number 2, 25 mm diameter) were acquired from VWR. The heterobifunctional linkers NHS-azide (#88902) and NHS-biotin (#20217) were purchased from Thermo Fisher Scientific. Ascorbic acid (>99.0%) and 96-well plates were purchased from Fisher Chemical & Scientific. Dimethylformamide (DMF) (>99.5%), dimethyl sulfoxide (99.5%) and sodium bicarbonate (99.0%) were acquired from EMD chemicals. Sulfuric acid was acquired from Avantor Performance Materials. Ethyl alcohol (EtOH) (200 proof) was purchased from Decon Labs. 3-Aminopropyltriethoxysilane and CH 3 (CH 2 CH 2 O) 9-12 (CH 2 ) 3 Si(OCH 3 ) 3 (mPEG) were acquired from Gelest. Unless otherwise stated, all the other starting materials and reagents were purchased from Sigma-Aldrich and used without further purification. All buffers were made with Nanopure water (18.2 MΩ) and passed through a 0.2 μm filtration system. How to cite this article: Zhang, Y. et al. DNA-based digital tension probes reveal integrin forces during early cell adhesion. Nat. Commun. 5:5167 doi: 10.1038/ncomms6167 (2014).